miR-1 and miR-206 target different genes to have opposing roles during angiogenesis in zebrafish embryos As miR-1 and miR-206 share identical seed sequences, they are commonly speculated to target the same gene. Here, we identify an mRNA encoding seryl-tRNA synthetase (SARS), which is targeted by miR-1, but refractory to miR-206 . SARS is increased in miR-1 -knockdown embryos, but it remains unchanged in the miR-206 knockdown. Either miR-1 knockdown or sars overexpression results in a failure to develop some blood vessels and a decrease in vascular endothelial growth factor Aa (VegfAa) expression. In contrast, sars knockdown leads to an increase of VegfAa expression and abnormal branching of vessels, similar to the phenotypes of vegfaa- overexpressed embryos, suggesting that miR-1 induces angiogenesis by repressing SARS. Unlike the few endothelial cells observed in the miR-1 -knockdown embryos, knockdown of miR-206 leads to abnormal branching of vessels accompanied by an increase in endothelial cells and VegfAa. Therefore, we propose that miR-1 and miR-206 target different genes and thus have opposing roles during embryonic angiogenesis in zebrafish. MicroRNAs ( miRNA s) are single-stranded RNA molecules, about 19–30 nucleotides (nt) in length, which repress the expression of their target genes through binding mRNAs at specific sequences. They control gene expression at post-translational level by various mechanisms, such as decay of mRNAs and blockage of translation [1] , [2] , [3] . Bioinformatics studies indicate that expressions of 30~50% of human genes are probably controlled by miRNA s [4] , [5] . Therefore, to understand the exact relationship between genes and their functions in embryos, it is necessary to clearly identify the target genes of specific miRNA s at particular developmental stages. miR-1 ( miR-1-1 and miR-1-2 ) and miR-206 are known as highly conserved miRNA s which share common expression in the muscles of organisms ranging from Caenorhabditis elegans to human [6] . However, miR-1-1, miR-1-2 and miR-206 are located at three different chromosomal regions, including 20q13.33, 18q11.2 and 6p12.2, respectively, in the human genome [7] . More specifically, although miR-1-1 locates at the intron of the C20orf166 gene, miR-1-2 locates at the intron of the Mindbomb gene, and miR-206 locates in the intergenic region [8] , [9] . Moreover, miR-1 and miR-206 have different pre- miRNA sequences, and they differ by four nt at mature miRNA [7] . It is also reported that miR-1 and miR-206 have different regulatory pathways. For example, overexpression of Myf5 and Myogenin in the neural tube can induce ectopic expressions of miR-1 and miR-206 , whereas overexpression of Myod can induce only miR-1 (ref. 6 ). miR-1 and miR-206 have different regulatory functions within the dystrophin/nNOS pathway [10] . These facts suggest that miR-1 and miR-206 may have different roles in gene regulation. Yet, as miR-1 and miR-206 share identical seed sequence, the results of any given bioinformatics search would predict the same target genes. Consequently, miR-1 and miR-206 are commonly speculated to have identical biological functions and are therefore considered to act conjointly as a single regulator termed as miR-1/206 . For example, miR-1/206 regulates connexin43 expression during skeletal muscle development [11] . miR-1/206 can repress vascular endothelial growth factor Aa gene ( vegfaa ) expression [12] . Therefore, whether miR-1 and miR-206 act separately to regulate different genes or act together to regulate the same genes remains controversial. In vitro studies suggested that miR-1 and miR-206 promote myoblast differentiation [7] . In zebrafish, miR-1 and miR-206 function in muscle gene expression and regulate sarcomeric actin organization [13] . Moreover, many factors, such as Seryl-transfer RNA synthetase (SARS) [14] and fibroblast growth factor signalling [15] , [16] , mediate Vegf expression in somites during embryogenesis. Nakasa et al. [17] reported that miR-1, -133 and -206 in muscle enhance angiogenesis during muscle regeneration. In contrast, Stahlhut et al. [12] found that miR-1/206 in muscle negatively regulates developmental angiogenesis through the repression of VegfAa expression. As no consensus has thus far been reached with respect to the regulatory function(s) of miR-1/206 , we conducted a more intensive examination of the molecular mechanism underlying the activity of these muscle-specific miRNA s in modulating angiogenesis during zebrafish embryonic development. To accomplish this, we employed the l abelled m iRNA p ull-down (LAMP) assay system [18] to obtain the target genes specific for miR-1 and miR-206 . Here, we found the endogenous sars -3′-untranslated region ( sars -3′UTR) target sequence (outside of seed) is refractory to miR-206 targeting, despite additional miR-206 complementarity. Instead, sars -3′UTR target sequence is specifically targeted by miR-1. Additionally, the vegfaa -3′UTR is only targeted by miR-206 but not miR-1 . Therefore, miR-1 and miR-206 act as independent upstream regulators, increasing or decreasing vegfaa expression, respectively, to ultimately have opposing roles in zebrafish angiogenesis. Our work points to specificity constraints that depend on the target sequence outside of the seed of miR-1 and miR-206 . Identification of putative target genes of mature miR-1 Using the LAMP assay system and microarray analysis, we have previously searched all the putative target genes of mature miR-1 (ref. 18 ). Here, we went further to focus on the candidate genes which are expressed in the muscle during zebrafish embryogenesis. The 3′UTR of these candidate genes for all 7-mer and 8-mer sequences complementary to zebrafish miR-1 seeds were searched by using RNAhybrid software [19] . Among 302 putative target genes for miR-1 , 88 are categorized as muscle-specific genes. We selected eight of them to perform luciferase ( luc ) assays. These 3′UTR cDNAs were individually cloned and engineered to fuse at the downstream of luc reporter gene and transfected together with miR-1 into cell lines C2C12 and HEK293T. Among them, the S-adenosylhomocysteine hydrolase gene was equally regulated by miR-1 and miR-206 , whereas eukaryotic translation initiation factor 2 subunit 1 alpha gene was neither regulated by miR-1 nor miR-206 ( Supplementary Fig. S1 ). Interestingly, as the luc activity was repressed in the construct containing 3′UTR of succinate-CoA ligase gene ( suclg1 ) and sars , they were determined to be targets of miR-1 with high potential ( Supplementary Fig. S1 ). Unexpectedly, we found that sars and suclg1 were regulated by miR-1 and that the spatiotemporal expressions of suclg1 and sars-mRNA were all detected in the somites of embryos at 20, 24 and 48 hours post-fertilization (hpf; Supplementary Fig. S1 ). As the luc assay demonstrated that sars was repressed effectively by miR-1 , we chose sars to perform the following experiments in more detail. The sars -mRNA is bound and regulated by miR-1 only The 3′UTRs of zebrafish, mouse and human sars were individually cloned and fused at the downstream of luc reporter gene ( Fig. 1a ). After these constructs were transfected separately, together with miR-1 , into human HEK293T cells, the luc activity was significantly decreased by 42% and 35% in the constructs containing zebrafish and human sars -3′UTRs, respectively ( Fig. 1b ). Similarly, in mouse C2C12 cells, the luc activity was significantly decreased by 47% and 36% in the construct containing zebrafish and mouse sars -3′UTRs, respectively ( Fig. 1b ), suggesting that miR-1 can bind to sars -3′UTR, resulting in the reduction of reporter activity. However, the luc activities fused with sars -3′UTRs from zebrafish and mouse remained unchanged when each construct was cotransfected with miR-206 into C2C12 cells ( Fig. 1c ), suggesting that sars -3′UTR is specifically bound by miR-1 , but not by miR-206 . 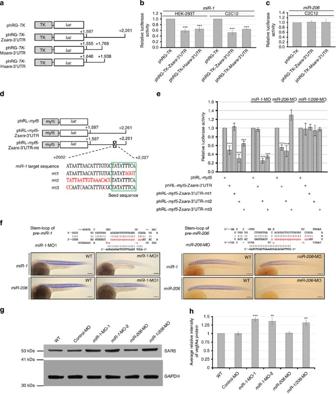Figure 1: OnlymiR-1specifically inhibitssarsexpressionin vitroandin vivo. (a) Diagrams of thelucreporter constructs containingsars-3′UTRs from different species such as zebrafish (Z); mouse (M) and human (H). (b) Histograms presented thelucactivity obtained from HEK-293T and C2C12 cells whenmiR-1was co-transfected with plasmids as indicated. The phRL-myf5vector served as a control group, and itslucactivity was set to 1. (c) Histograms presented thelucactivity obtained from C2C12 cells whenmiR-206was co-transfected with plasmids as indicated. The phRL-myf5vector served as a control group, and itslucactivity was set to 1. (d) Diagrams of thelucreporter constructs containing Wt and mutatedsars-3′UTRs. The mutated sequence was labelled with red. The seed sequence was blocked with green. (e) Histograms presented thelucactivity obtained from embryos at 24 hpf. Plasmid phRL-myf5vector served as a control group, and itslucactivity was set to 1. Thelucactivity assay in panels (b), (c) and (e) are calculated from three independent experiments and presented as mean±s.d. (n=3). Student’st-test was used to determine significant differences between each construct and control within each group (***P<0.005). (f) The sequences of pre-miR-1and pre-miR-206were aligned tomiR-1-MO1 andmiR-206-MO, respectively, as shown. WISH ofmiR-1andmiR-206in WT,miR-1-MO1- andmiR-206-MO-injected embryos was examined at 30 hpf. Scale bar presents 300 μm. (g) The patterns of SARS protein in WT and embryos injected with control-MO (8 ng),miR-1-MO1 (8 ng),miR-1-MO2 (8 ng),miR-206-MO (8 ng) andmiR-1/206-MO (8 ng) at 48 hpf by western blot analysis. GAPDH was used as an internal control. (h) Statistical analysis of the average relative intensity of SARS protein from each group was presented. Data are calculated from three independent experiments and presented as mean±s.d. (n=3). Student’st-test was used to determine significant differences between each construct and control within each group (***P<0.005 and **P<0.01). Figure 1: Only miR-1 specifically inhibits sars expression in vitro and in vivo . ( a ) Diagrams of the luc reporter constructs containing sars -3′UTRs from different species such as zebrafish (Z); mouse (M) and human (H). ( b ) Histograms presented the luc activity obtained from HEK-293T and C2C12 cells when miR-1 was co-transfected with plasmids as indicated. The phRL- myf5 vector served as a control group, and its luc activity was set to 1. ( c ) Histograms presented the luc activity obtained from C2C12 cells when miR-206 was co-transfected with plasmids as indicated. The phRL- myf5 vector served as a control group, and its luc activity was set to 1. ( d ) Diagrams of the luc reporter constructs containing Wt and mutated sars -3′UTRs. The mutated sequence was labelled with red. The seed sequence was blocked with green. ( e ) Histograms presented the luc activity obtained from embryos at 24 hpf. Plasmid phRL- myf5 vector served as a control group, and its luc activity was set to 1. The luc activity assay in panels ( b ), ( c ) and ( e ) are calculated from three independent experiments and presented as mean±s.d. ( n =3). Student’s t -test was used to determine significant differences between each construct and control within each group (*** P <0.005). ( f ) The sequences of pre- miR-1 and pre- miR-206 were aligned to miR-1 -MO1 and miR-206 -MO, respectively, as shown. WISH of miR-1 and miR-206 in WT, miR-1 -MO1- and miR-206 -MO-injected embryos was examined at 30 hpf. Scale bar presents 300 μm. ( g ) The patterns of SARS protein in WT and embryos injected with control-MO (8 ng), miR - 1 -MO1 (8 ng), miR - 1 -MO2 (8 ng), miR-206 -MO (8 ng) and miR-1/206 -MO (8 ng) at 48 hpf by western blot analysis. GAPDH was used as an internal control. ( h ) Statistical analysis of the average relative intensity of SARS protein from each group was presented. Data are calculated from three independent experiments and presented as mean±s.d. ( n =3). Student’s t -test was used to determine significant differences between each construct and control within each group (*** P <0.005 and ** P <0.01). Full size image We further studied whether sars -3′UTR is only regulated by endogenous miR-1 in zebrafish embryos. To accomplish this, we constructed plasmid phRL- myf5 -Z sars -3′UTR, in which a zebrafish sars -3′UTR was fused with luc reporter and driven by zebrafish myf5 promoter to serve as a control group ( Fig. 1d,e ). A mutated plasmid, phRL- myf5 -Z sars -3′UTR-mt1, was also constructed, in which the predicted target sites for miR-1 , that is, TTCA located at +2,024 to +2,027 nt, were mutated into AGGT ( Fig. 1d ). Compared with the control group, the luc activity of the embryos injected with phRL- myf5 -Z sars -3′UTR was greatly decreased by 55%, whereas that of embryos injected with phRL- myf5 -Z sars -3′UTR-mt1 remained unchanged ( Fig. 1e ), indicating that mutation of miR-1 target sequences resulted in abolishing the repression of miR-1 , allowing it to bind and silence sars, both in vitro and in vivo. In addition, we designed miR-1 -MO1, miR-1 -MO2, miR-206- MO and miR-1/206- MO, which simultaneously knockdown both miR-1 and miR-206 , as well as control-MO, for further experiments ( Supplementary Fig. S3 ). Whole-mount in situ hybridization (WISH) showed that the miR-1 was only absent in the miR-1- MO1- and miR-1 -MO2-injected embryos, whereas miR-206 was only absent in the miR-206- MO-injected embryos ( Fig. 1f and Supplementary Fig. S3 ), indicating that the MOs we used were specific for miR-1 and miR-206 individually. When miR-1 was knocked down by injection of miR-1 -MO1, the luc activity of embryos injected with phRL- myf5 -Z sars -3′UTR was close to that of control phRL- myf5- injected embryos ( Fig. 1e ), suggesting that the endogenous miR-1 was reduced by introducing miR-1 -MO1 and lost its ability to silence phRL- myf5 -Z sars -3′UTR in embryos. When embryos were injected with phRL- myf5 -Z sars -3′UTR plus miR-206 -MO, luc activity continued to decrease ( Fig. 1e ), indicating that miR-206 was not involved in silencing the injected phRL- myf5 -Z sars -3′UTR in embryos. These findings further suggest that sars -3′UTR is regulated by endogenous miR-1 , not miR-206 , in zebrafish embryos. On the basis of the prediction of bioinformatics software, such as RNAhybrid [19] , the complementarity between the target sequence (+2,002 to +2,027) and each miRNA is shown in Supplementary Fig. S4 . To demonstrate that both seed and sequences in the neighbourhood of the seed are involved in the specificity of miRNA differential targeting, we constructed two plasmids: phRL- myf5 -Zsars-3′UTR-mt2 and phRL- myf5 -Zsars-3′UTR-mt3. The first plasmid contains a mutated sequence in the 3′UTR of sars whose miR-1 target sequence outside the seed is altered, whereas the second plasmid contains a mutated sequence in the 3′UTR of sars whose miR-1 target site is altered such that a base pair extensively matches that of miR-206. Compared with control, the luc activity was also greatly reduced in embryos injected with phRL- myf5 -Zsars-3′UTR-mt2 ( Fig.1e ). However, this reduction could not be restored by knocking down either miR-1 or miR-206 ( Fig. 1e ), indicating that the mutated sequence outside the seed sequence of miR-1 leads to failure in selecting a specific target for miR-1 . Furthermore, the luc activity of dual miR-1 / miR-206 knockdown embryos was close to that of embryos injected with phRL- myf5 (control), embryos injected with phRL- myf5 -Z sars -3′UTR and embryos injected with mt2 mutated constructs ( Fig. 1e ). Thus, both miR-1 and miR-206 target the same site, in turn reducing luc activity ( Fig. 1e ). These data indicates that a target outside the seed sequence of miR-1 is a critical factor related to the selection of either miR-1 or miR-206 targeting. Importantly, when we injected embryos with phRL- myf5 -Zsars-3′UTR-mt3 altered in the manner suggested above, the luc activity was still reduced in miR-1- knockdown embryos, but fully restored in miR-206 - and miR-1/206 -knockdown embryos, compared with control group ( Fig. 1e ). These data indicate that a difference of only four nt between miR-1 and miR-206 becomes a sequence that is determinative of the differential targeting between miR-1 and miR-206 . We also analysed the protein levels of SARS in embryos injected with control-MO, miR-1 -MO1, miR-1 -MO2, miR-206 -MO and miR-1/206 -MO. Results showed that the SARS protein level was increased in embryos injected miR-1 -MO1 (average relative intensity (ari)±standard deviation (s.d.) was 1.42±0.05), miR-1 -MO2 (ari±s.d.=1.36±0.10) and miR-1/206 -MO (ari±s.d.=1.32±0.09) relative to that of embryos injected with control-MO (ari±s.d.=0.99±0.05). Similar to the luc data, embryos injected with miR-206 -MO did not show any change in SARS protein level (ari±s.d.=1.02±0.05) ( Fig. 1g,h ). Together, we concluded that miR-1, but not miR-206, regulates sars expression during zebrafish development. miR-1 promotes angiogenesis through reducing SARS protein In zebrafish, the non-canonical activity of SARS in somites is involved in the vascular development through modulating the expression of vegfaa [14] , [20] . Our data showed that knockdown of miR-1 can increase SARS protein level in embryos, suggesting that excessive SARS may, in turn, repress vegfaa expression to affect angiogenesis. To prove this hypothesis, we performed either knockdown of miR-1 or overexpression of sars -mRNA and analysed vascular development using the transgenic line Tg(fli-EGFP) y1 whose endothelial cells are labelled by enhanced green fluorescent protein (EGFP). In the uninjected control embryos during 30–72 hpf, we observed that (1) the blood vessels crossed the transverse myoseptum to form parachordal vessels (PAVs) and (2) most intersegmental vessels (ISVs) grew rostrally from dorsal aorta and then extended caudally, following the chevron-like contours of the somites to reach the dorsal–lateral surface where tubes from adjacent ISVs fused to form dorsal longitudinal anastomotic vessels ( Fig. 2a ). However, in the miR-1 morphants ( Fig. 2b ), sars -mRNA-injected embryos ( Fig. 2c ), and T429A- mRNA-injected embryos, a sars mutated form absent in serine binding ( Fig. 2d ) [14] , we found that (1) the development of ISVs was terminated and stacked at the myoseptal midpoint during 30 hpf, (2) ISVs were misdirected and appeared laterally asymmetrical, (3) PAVs grew slowly, and, finally, (4) PAV and DLAV were incompletely formed during 48 and 72 hpf. These data indicate that either the overexpression of SARS or the induction of SARS expression by introducing miR-1- MO1 causes the absence of developing blood vessels in embryos. In addition, the miR-1- MO1 phenotype could be rescued by coinjecting an excessive amount of sars -MO ( Fig. 2b versus f ). Unlike the miR-1 -morphants, which were unable to continue development of blood vessels, the trunk vasculatures were almost completely formed in miR-1 / sars -MO-injected embryos. Ectopic sprouting of the tip cells was detected (white arrowheads of Fig. 2f ), which was similar to the phenotypes of sars morphants. On the other hand, either knockdown of sars by injection of sars -MO ( Fig. 2e ) or overexpression of VegfAa by injection of vegfaa -mRNA ( Fig. 2i ) led to abnormally branched blood vessels among ISVs in trunk during 30–72 hpf ( Fig. 2e,h ). Furthermore, the phenotype was specific to miR-1 downregulation, as evidenced by the following observations. First, the defects could be phenocopied by coinjection of miR-1 -MO1 and p53 -MO. Second, the defects were not seen in either standard control MO-injected embryos or miR-1- 5mis-MO-injected embryos ( Supplementary Fig. S5 ). Our data demonstrated that miR-1 induces angiogenesis through repressing SARS expression during embryonic development. 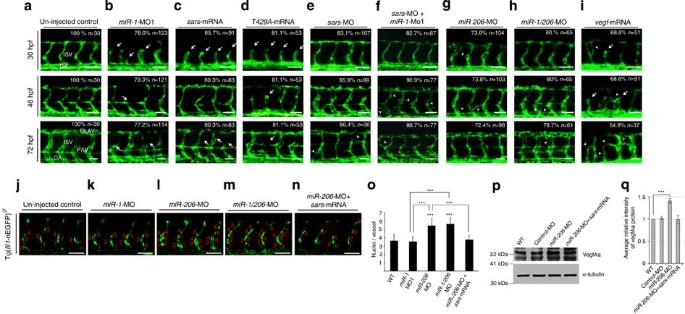Figure 2: Distinct functions ofmiR-1andmiR-206in angiogenesis during zebrafish embryonic development. (a) Embryos derived from transgenic lineTg(fli1:EGFP) without treatment served as control. These embryos were injected with (b) 8 ng ofmiR-1-MO1, (c) 300 pg ofsars-mRNA, (d) 300 pg ofT429A-mRNA, (e) 4 ng ofsars-MO, (f) 6 ng ofmiR-1-MO1 plus 3 ng ofsars-MO, (g) 8 ng ofmiR-206-MO, (h) 8 ng ofmiR-1/206-MO and (i) 50 pg ofvegf121-mRNA. All the embryos were observed at 30, 48 and 72 hpf. (j–n) Embryos derived from lineTg(fli-nGFP)y7without treatment served as control. Each nucleus was marked with a number. The total number of nuclei was counted in (j) uninjected control embryos and in embryos injected with (k)miR-1-MO1, (l)miR-206-MO, (m)miR-1/206-MO or (n)miR-206-MO/sars-mRNA. (o) Statistical analyses of the average number of nuclei per ISV amongmiR-1-MO1-,miR-206-MO-,miR-1/206-MO- andmiR-206-MO/sars-mRNA-injected embryos at 30 hpf were indicated. Data are calculated from three independent experiments and presented as mean±s.d. (n=3). (p) The patterns of SARS protein in WT and embryos injected with control-MO,miR-206-MO andmiR-206-MO/sars-mRNA at 48 hpf, by western blot analysis. α-tubulin was used as an internal control. (q) Statistical analysis of the average relative intensity (ari) of SARS protein level from each group was presented. Data are calculated from three independent experiments and presented as mean±s.d. (n=3). Student’st-test was used to determine significant differences between each group (***P<0.005). ISV, intersegmental vessel; DLAV, dorsal longitudinal anastomotic vessel; PAV, parachordal vessel; DA, dorsal aorta; scale bar, 100 μm. Figure 2: Distinct functions of miR-1 and miR-206 in angiogenesis during zebrafish embryonic development. ( a ) Embryos derived from transgenic line Tg ( fli1:EGFP ) without treatment served as control. These embryos were injected with ( b ) 8 ng of miR - 1 -MO1, ( c ) 300 pg of sars -mRNA, ( d ) 300 pg of T429A -mRNA, ( e ) 4 ng of sars -MO, ( f ) 6 ng of miR - 1 -MO1 plus 3 ng of sars -MO, ( g ) 8 ng of miR - 206 -MO, ( h ) 8 ng of miR-1/206 -MO and ( i ) 50 pg of vegf 121-mRNA. All the embryos were observed at 30, 48 and 72 hpf. ( j – n ) Embryos derived from line Tg(fli-nGFP) y7 without treatment served as control. Each nucleus was marked with a number. The total number of nuclei was counted in ( j ) uninjected control embryos and in embryos injected with ( k ) miR-1 -MO1, ( l ) miR-206 -MO, ( m ) miR-1/206- MO or ( n ) miR-206 -MO/ sars -mRNA. ( o ) Statistical analyses of the average number of nuclei per ISV among miR-1 -MO1-, miR-206 -MO-, miR-1/206 -MO- and miR-206 -MO/ sars -mRNA-injected embryos at 30 hpf were indicated. Data are calculated from three independent experiments and presented as mean±s.d. ( n =3). ( p ) The patterns of SARS protein in WT and embryos injected with control-MO, miR-206 -MO and miR-206 -MO /sars- mRNA at 48 hpf, by western blot analysis. α-tubulin was used as an internal control. ( q ) Statistical analysis of the average relative intensity (ari) of SARS protein level from each group was presented. Data are calculated from three independent experiments and presented as mean±s.d. ( n =3). Student’s t -test was used to determine significant differences between each group (*** P <0.005). ISV, intersegmental vessel; DLAV, dorsal longitudinal anastomotic vessel; PAV, parachordal vessel; DA, dorsal aorta; scale bar, 100 μm. Full size image miR-206 inhibits angiogenesis during zebrafish embryogenesis Although Stahlhut et al. [12] reported that miR-1/206 in muscle negatively regulates developmental angiogenesis, it is unclear whether miR-206 has an independent role in angiogenesis. To address this question, we employed MOs which can specifically knockdown miR-1 or/and miR-206 ( Fig. 1f ). Embryos injected with miR-206- MO ( Fig. 2g ) or miR-1/206 -MO ( Fig. 2h ) led to abnormally branched blood vessels among ISVs in trunk during 30–72 hpf. In addition, similar to the uninjected control embryos ( Fig. 2j ), three to four endothelial cells were observed in the Tg(fli-nuclearGFP) y7 embryos injected with miR-1- MO1 during 24–28 hpf ( Fig. 2k ). However, either single knockdown of miR-206 ( Fig. 2l , Supplementary Fig. S6 ) or double knockdown of miR-1/206 ( Fig. 2m ) led to the abnormal branching in trunk blood vessels accompanied by a significant increase in the number of endothelial cells to as many as seven at the same stage ( Fig. 2m,o ). The result for miR-1/206 -MO-injected embryos was consistent with Stahlhut et al. [12] who reported that the number of endothelial cells in miR-1/206 -MO-injected embryos was increased. Live imaging analyses of control-MO, miR-1- MO1- and miR-206- MO-injected embryos derived from line Tg(fli-nuclearGFP) y7 revealed that the increase of cell number in the miR-206 -knockdown embryos resulted from enhanced endothelial cell migration as well as elevated cell proliferation, once endothelial cells entered the intersomitic region. In contrast, knockdown of miR-1 had no effect on endothelial cell behaviour. Instead, angiogenesis was repressed in embryos without miR-1 . In addition, overexpression of sars -mRNA could rescue the pro-angiogenic effects caused by injection of miR-206 -MO ( Fig. 2n,o ), indicating that changes in SARS protein level can influence miR-206 -mediated anti-angiogenic effects. Furthermore, we demonstrated that the protein level of VegfAa was increased (ari±s.d.=1.41±0.06) in the embryos injected with miR-206 -MO, compared with that of control-MO-injected embryos (ari±s.d.=1.02±0.04; Fig. 2p,q ). Importantly, compared with wild-type (WT) embryos and miR-206 morphants, we found that VegfAa was not excessively expressed in embryos injected with miR-206 -MO plus sars- mRNA (ari±s.d.=0.99±0.09). These results indicated that the increase of VegfAa resulting from the suppression of miR-206 can be rescued by the addition of sars- mRNA. To examine differential regulation of vegfaa by miR-1 and miR-206 , we used the luc reporter construct containing WT and mutated vegfaa -3′UTR [12] . Results showed that the luc activity of the mutated vegfaa reporter whose seed sequence CATTCC had been mutated to CTAACC (Z vegf-3′UTR -mt1) was greatly increased ( Fig. 3 ). Coinjection of the WT vegfaa- 3′UTR reporter plus miR-206 -MO restored the reduced luciferase expression to a level similar to that of embryos injected with mutant reporter ( Fig. 3 ). However, coinjection of the WT vegfaa- 3′UTR reporter plus miR-1 -MO1 did not change the luc activity ( Fig. 3 ), suggesting that only miR-206 , but not miR-1 , specifically targets vegfaa- 3′UTR to mediate vegfaa expression. 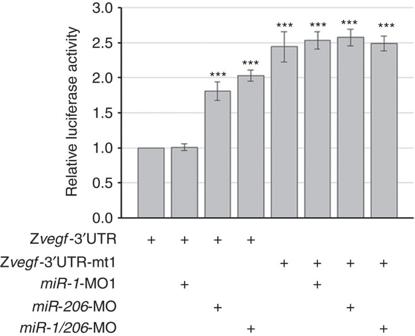Figure 3: The zebrafishvegfaamRNA is regulated differently bymiR-1andmiR-206. Histograms presented thelucactivity obtained from zebrafish embryos at 24 hpf. Plasmid pCS2+-Zvegf-3′UTR served as a control group, and itslucactivity was set to 1. Thelucactivity assay are calculated from three independent experiments and presented as mean±s.d. (n=3). Student'st-test was used to determine significant differences between each construct and control within each group (***P<0.005). Figure 3: The zebrafish vegfaa mRNA is regulated differently by miR-1 and miR-206 . Histograms presented the luc activity obtained from zebrafish embryos at 24 hpf. Plasmid pCS2 + -Z vegf -3′UTR served as a control group, and its luc activity was set to 1. The luc activity assay are calculated from three independent experiments and presented as mean±s.d. ( n =3). Student's t -test was used to determine significant differences between each construct and control within each group (*** P <0.005). Full size image Together, the above results indicated that miR-1 and miR-206 have distinctly different roles in the development of the ISV. Specifically, miR-1 positively affects angiogenesis through sars regulation, whereas miR-206 negatively affects angiogenesis independent of sars regulation. miR-1 represses SARS through direct targeting of sars- mRNA To further confirm that sars- 3′UTR is a direct target of miR-1 , we employed a target protector morpholino (TP-MO) [12] , [21] , [22] , which is complementary to the miR-1 target site ( Fig. 4a ), resulting in the inhibition of miR-1 targeting on sars -3′UTR. We also constructed two plasmids in which the downstream of EGFP reporter was fused with either the full length of WT sars -3′UTR or the mutated sequence of sars -3′UTR. When we injected egfp -mRNA containing either WT sars -3′UTR or mutated sars -3′UTR into the one-cell stage, the GFP signal was observed in embryos at 24 hpf. The GFP signal was observed throughout the embryo in the positive control group whose embryos were injected with egfp -mRNA plus control-MO ( Fig. 4b ), However, a significant reduction in GFP signal was observed in the trunk muscles of negative control group whose embryos were injected with egfp -mRNA containing WT sars -3′UTR by the presence of endogenous miR-1 ( Fig. 4c ). Interestingly, we found that the GFP signal was not reduced in the trunk muscles of embryos injected with egfp -mRNA containing either the mutated sars -3′UTR plus control-MO ( Fig. 4d ) or WT sars -3′UTR plus sars -TP-MO ( Fig. 4e ), suggesting that miR-1 silencing is abolished when the miR-1 -target sequence on sars -3′UTR is blocked by sars -TP-MO. Furthermore, we found that injection of WT sars -3′UTR plus miR-1 -MO1 could restore the reduced GFP signal caused by miR-1 knockdown ( Fig. 4f ). However, injection of WT sars -3′UTR plus miR-206 -MO could not restore the reduced GFP signal ( Fig. 4g ). In addition, western blot analysis demonstrated that the SARS protein level was increased (ari±s.d.=1.41±0.06 versus ari±s.d.=1.01±0.04 for control-MO-injected embryos), whereas the VegfAa protein level was decreased (ari±s.d.=0.39±0.09 versus ari±s.d.=1.04±0.02 for control-MO-injected embryos) in sars -TP-MO-injected embryos ( Fig. 4h,i ). Therefore, when the miR-1 target site is blocked by sars -TP-MO, sars -mRNA can stabilize, resulting in the translation of more SARS, which in turn, reduces VegfAa. 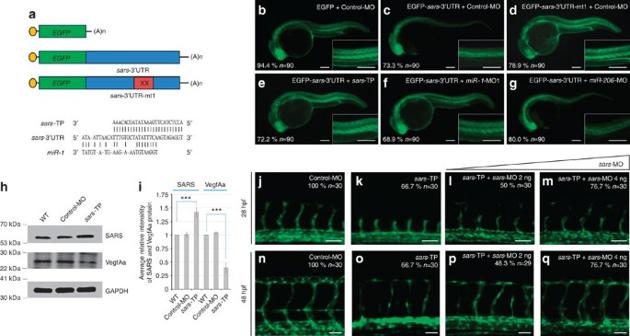Figure 4: Using morpholino target protector (TP) to show thatmiR-1represses zebrafishsars-3′UTR. (a) Sequence of the target site, cognatesars-TP-MO (sars-TP), andmiR-1were indicated. The full length ofsars-3′UTR was inserted downstream of an EGFP expression vector. (b) In the control group, the GFP signal was observed throughout the embryos injected withegfp-mRNA plus control-MO. (c) The GFP signal in truck somites, shown at right lower corner, was greatly reduced in embryos injected with control-MO plusegfp-mRNA containing WTsars-3′UTR. (d) The GFP signal in truck somite was restored when themiR-1target site onsars-3′UTR was mutated. (e) The GFP signal in truck somite was also restored in embryos injected with EGFP-WTsars-3′UTR plussars-TP-MO. (f) The reduced GFP caused by EGFP-sars-3′UTR could be restored by coinjection ofmiR-1-MO1. (g) The reduced GFP caused by EGFP-sars-3′UTR could not be restored by coinjection ofmiR-206-MO. (h) Western blot analysis to detect the proteins of SARS and VegfAa in the WT, control-MO-injected andsars-TP-MO-injected embryos at 48 hpf. (i) The statistical analyses of the average relative intensities of SARS and VegfAa performed on densitometry from WT, control-MO-injected andsars-TP-MO-injected embryos after three independent experiments. Data are presented as mean±s.d. (n=3). Student'st-test was used to determine significant differences between each construct and control within each group (***P<0.005). GAPDH served as an internal control. (j–q) Embryos derived from lineTg(fli1:EGFP) were injected with materials as indicated, and ISV patterns were observed at 28 and 48 hpf. Scale bar: (b–g) 300 μM; (j–q) 100 μM. Figure 4: Using morpholino target protector (TP) to show that miR-1 represses zebrafish sars -3′UTR. ( a ) Sequence of the target site, cognate sars -TP-MO ( sars -TP), and miR-1 were indicated. The full length of sars -3′UTR was inserted downstream of an EGFP expression vector. ( b ) In the control group, the GFP signal was observed throughout the embryos injected with egfp -mRNA plus control-MO. ( c ) The GFP signal in truck somites, shown at right lower corner, was greatly reduced in embryos injected with control-MO plus egfp -mRNA containing WT sars -3′UTR. ( d ) The GFP signal in truck somite was restored when the miR-1 target site on sars -3′UTR was mutated. ( e ) The GFP signal in truck somite was also restored in embryos injected with EGFP-WT sars -3′UTR plus sars -TP-MO. ( f ) The reduced GFP caused by EGFP- sars -3′UTR could be restored by coinjection of miR-1 -MO1. ( g ) The reduced GFP caused by EGFP- sars -3′UTR could not be restored by coinjection of miR-206 -MO. ( h ) Western blot analysis to detect the proteins of SARS and VegfAa in the WT, control-MO-injected and sars -TP-MO-injected embryos at 48 hpf. ( i ) The statistical analyses of the average relative intensities of SARS and VegfAa performed on densitometry from WT, control-MO-injected and sars -TP-MO-injected embryos after three independent experiments. Data are presented as mean±s.d. ( n =3). Student's t -test was used to determine significant differences between each construct and control within each group (*** P <0.005). GAPDH served as an internal control. ( j – q ) Embryos derived from line Tg(fli1:EGFP ) were injected with materials as indicated, and ISV patterns were observed at 28 and 48 hpf. Scale bar: ( b – g ) 300 μM; ( j – q ) 100 μM. Full size image To examine the specific effect of sars -TP-MO in vivo on sars- mRNA, we injected sars -TP-MO into embryos derived from transgenic line Tg(fli-nGFP) y7 and monitored the development of ISVs labelled by GFP. Compared with control group, the angiogenesis of embryos-injected sars -TP-MO was repressed ( Fig. 4j versus k ). This phenotype recapitulated the vascular defect observed in the miR-1 knockdown embryos ( Fig. 4k versus 2b ). However, this phenotype could be rescued by coinjecting an excessive amount of sars -MO ( Fig. 4k versus l, m ; Fig. 4o versus p, q ). Unlike the miR-1 morphants which were unable to continue development of blood vessels, the trunk vasculatures were almost completely formed in sars- TP/ sars -MO-injected embryos. Ectopic sprouting of the tip cells was detected, which was similar to the phenotypes of sars morphants. The miR-1 /SARS pathway modulates vegfaa expression This miR-1 /SARS regulatory pathway is different from the miR-1/206/ Vegf regulatory pathway proposed by Stahlhut et al. [12] in that they observed the promotion of vegfaa expression in miR-1/206 double knockdown zebrafish embryos. However, although we have demonstrated that miR-1 promotes angiogenesis through silencing SARS, it is unclear whether such effect is direct or whether the miR-1 /SARS regulatory pathway acts as an upstream modulator of vegfaa expression to, in turn, promote angiogenesis in somitic cells. To address this question, we quantified vegfaa -mRNA in 48 hpf embryos injected separately with miR-1 -MO1 and sars -mRNA. Results showed that the expression of vegfaa- mRNA was greatly reduced in the miR-1 morphants and sars -overexpressed embryos ( Fig. 5a ). Second, western blot analysis showed that VegfAa was also reduced in miR-1 morphants, whereas VegfAa was increased both in miR-206- MO- and miR-1/206- MO-injected embryos ( Fig. 5b ). Similar results were obtained in the mammalian system because we found that overexpression of miR-1 in cell line C2C12 caused a 46% decrease of SARS, and a 29% increase of VegfAa protein, whereas overexpression of mouse sars- mRNA caused a 41% increase of SARS and a 45% decrease of VegfAa ( Fig. 5c,d ). Thus, we concluded that VegfAa was reduced when miR-1 was absent, but that it was increased when SARS was absent, suggesting that miR-1 reduces SARS, which, in turn, results in the increase of VegfAa. In addition, as determined by enzyme-linked immunosorbent assay (ELISA), we found that the overexpression of pre- miR-1 in C2C12 cells caused a 45% increase of VegfAa expression ( Fig. 5e ), whereas, on the other hand, overexpression of SARS caused a 40% decrease of VegfAa expression ( Fig. 5e ), suggesting that the secretion of VegfAa from C2C12 cells can be affected by either miR-1 or SARS. We also observed that the nuclear content of SARS protein was increased by 28% and 75% in the knockdown of miR-1 and overexpression of SARS, respectively, during zebrafish embryogenesis ( Fig. 5f ). These data supported Xu et al. [20] who proved that SARS negatively regulates vegfaa transcription through entering the nucleus. Together, we proposed that miR-1 functions to reduce the protein level of SARS in somites in order to keep excessive SARS from entering the nucleus, which, in turn, promotes vegfaa expression in blood vessels. This fact is consistent between zebrafish in vivo study and mammalian in vitro study. 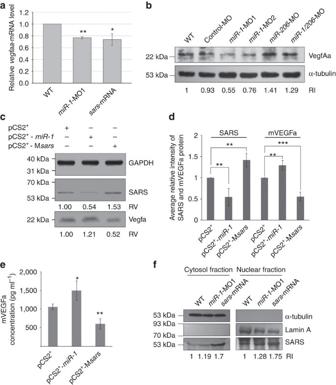Figure 5: Knockdown ofmiR-1and overexpression ofsarsresult in downregulating the expression ofvegfaa. (a) The statistical analysis of quantitative RT-PCR ofvegfaa-mRNA level in the embryos injected withmiR-1-MO1 (8 ng) andsars-mRNA (300 pg) at 48 hpf. The intensity ofvegfaa-mRNAs in WT served as control and was set as 1. Data are presented as mean±s.d. (n=3). Student’st-test was used to determine significant differences between each group (*P<0.05, **P<0.01). (b) Western blot analysis of VegfAa protein level in zebrafish embryos was presented. The relative intensities (RI) of VegfAa protein among WT, Control-MO-,miR-1-MO1-,miR-1-MO2-,miR-206-MO- andmiR-1/miR-206-MO-injected embryos were as indicated. The protein level of α-tubulin served as an internal control for loading amount of proteins. (c) Western blot analyses of total proteins extracted from cell line C2C12 which was individually transfected with pCS2+vector, pCS2+-miR-1and pCS2+-Msars(mousesarscDNA). The relative intensity (RI) of SARS and VegfAa proteins among pCS2+-, pCS2+-miR-1-and pCS2+-Msars-transfected cells were indicated. The protein level of GAPDH served as an internal control. (d) Statistical analyses of the average relative intensity (ari) of SARS and VegfAa proteins from each group were presented. Data are calculated from three independent experiments and presented as mean±s.d. (n=3). Student'st-test was used to determine significant differences between each group (**P<0.01, ***P<0.005). (e) ELISA to determine the amount of VegfAa secreted from C2C12 when pre-miR-1and SARS protein were overexpressed. Data are calculated from three independent experiments and presented as mean±s.d. (n=3). Student’st-test was used to determine significant differences between each group (*P<0.05, **P<0.01). The RI of mVegfa protein among in each group was as indicated. (f) Western blot analysis of SARS protein level in the cytosol fraction and nuclear fraction extracted from WT,miR-1-MO1- andsars-mRNA-injected embryos were as indicated. The protein levels of α-tubulin and Lamin A were used as internal control of cytosol fraction and nuclear fraction, respectively. Figure 5: Knockdown of miR-1 and overexpression of sars result in downregulating the expression of vegfaa . ( a ) The statistical analysis of quantitative RT-PCR of vegfaa -mRNA level in the embryos injected with miR-1 -MO1 (8 ng) and sars -mRNA (300 pg) at 48 hpf. The intensity of vegfaa -mRNAs in WT served as control and was set as 1. Data are presented as mean±s.d. ( n =3). Student’s t -test was used to determine significant differences between each group (* P <0.05, ** P <0.01). ( b ) Western blot analysis of VegfAa protein level in zebrafish embryos was presented. The relative intensities (RI) of VegfAa protein among WT, Control-MO-, miR - 1 -MO1-, miR - 1 -MO2-, miR-206 -MO- and miR - 1/miR-206 -MO-injected embryos were as indicated. The protein level of α-tubulin served as an internal control for loading amount of proteins. ( c ) Western blot analyses of total proteins extracted from cell line C2C12 which was individually transfected with pCS2 + vector, pCS2 + - miR-1 and pCS2 + -M sars (mouse sars cDNA). The relative intensity (RI) of SARS and VegfAa proteins among pCS2 + -, pCS2 + - miR-1- and pCS2 + -M sars- transfected cells were indicated. The protein level of GAPDH served as an internal control. ( d ) Statistical analyses of the average relative intensity (ari) of SARS and VegfAa proteins from each group were presented. Data are calculated from three independent experiments and presented as mean±s.d. ( n =3). Student's t -test was used to determine significant differences between each group (** P <0.01, *** P <0.005). ( e ) ELISA to determine the amount of VegfAa secreted from C2C12 when pre- miR-1 and SARS protein were overexpressed. Data are calculated from three independent experiments and presented as mean±s.d. ( n =3). Student’s t -test was used to determine significant differences between each group (* P <0.05, ** P <0.01). The RI of mVegfa protein among in each group was as indicated. ( f ) Western blot analysis of SARS protein level in the cytosol fraction and nuclear fraction extracted from WT, miR-1 -MO1- and sars -mRNA-injected embryos were as indicated. The protein levels of α-tubulin and Lamin A were used as internal control of cytosol fraction and nuclear fraction, respectively. Full size image Interestingly, we performed qPCR to quantify the expression levels of miR-1 and miR-206 in embryos from 12 to 32 hpf to determine any differences in the timing of expression levels of miR-1 and miR-206. Results showed that the expression level of miR-1 was gradually increased during 12–20 hpf. But, the value was dramatically increased from 20 to 32 hpf ( Supplementary Fig. S7A,B ). However, the expression level of miR-206 was insignificantly changed during these stages ( Supplementary Fig. S7A,B ). In addition, we determined miR-1 and miR-206 copy numbers at different developmental stages which are based on the relative value against the known copies in a genome sequence, such as U6 (refs 23 , 24 , 25 ). The relative copy number of miR-1 per 100 U6 was gradually increased during 12–20 hpf ( Supplementary Fig. S7C ). Particularly, the value was dramatically increased from 20 to 32 hpf ( Supplementary Fig. S7C ). In contrast, the relative copy number of miR-206 per 100 U6 was insignificantly changed during these stages ( Supplementary Fig. S7C ). Taken together, this evidence indicates that the amount of miR-1 is greatly increased from 20 to 32 hpf, whereas that of miR-206 remains insignificant throughout these stages of development. Moreover, the great increase of VegfAa during 24–30 hpf, which was reported by Liang et al. [26] , might be responsible for the continuous increase of miR-1 /SARS/VegfAa axis, but not miR-206 /VegfAa axis. Therefore, we can safely conclude that differences in the timing of repression of miR-1 and miR-206 occur during embryogenesis, suggesting, in turn, that the miR-1 /SARS/VegfAa pathway increasingly affects embryonic angiogenesis at late developmental stages in somitic cells. The non-canonical activity of SARS in somites is involved in vascular development by modulating the expression of vegfaa [14] . Xu et al. [20] identified a nuclear localization signal sequence embedded in the UNE-S domain at the carboxyl-terminus of SARS, which can help SARS enter the nucleus and repress vegfaa expression. In the present report, we found that miR-1 , but not miR-206 , can specifically repress SARS expression by targeting the 3′UTR of sars -mRNA. Our data also proved that either excessive expression of SARS or knockdown of miR-1 in zebrafish embryos can increase the amount of SARS entering the nucleus. The rescue experiment showed that knockdown of SARS in the miR-1 -MO1-injected embryos could rescue Se vessel defects induced by miR-1 -MO1. Therefore, it was proposed that miR-1 positively regulates VegfAa expression by limiting the amount of SARS protein in somites. Our data shows that, first, the vegfaa- 3′UTR is regulated differently by miR-1 and miR-206 ; second, overexpression of SARS can rescue the elevated numbers of endothelial cells caused by miR-206 knockdown; third, SARS is increased, but VegfAa is reduced, in miR-1- MO-injected embryos, whereas SARS remains unchanged, but VegfAa is increased, in miR-206- MO-injected embryos; and finally, SARS is a negative regulator of VegfAa. Therefore, we proposed that miR-1 has a regulatory role opposite to that of miR-206 through directly controlling the level of SARS protein, but indirectly controlling the level of VegfAa protein level, during zebrafish angiogenesis. That is, although the miR-1 /SARS regulatory pathway promotes embryonic angiogenesis by the upstream modulation of vegfaa , miR-206 has an anti-angiogenic role by directly controlling VegfAa protein level. We noticed that the similarity of angiogenic defects between those caused by miR-206 single knockdown embryos and miR-1/206 double knockdown embryos agrees with Stahlhut et al. [12] who reported that the number of endothelial cells in miR-1/206 -MO-injected embryos was increased. However, the angiogenic phenotypes caused by miR-1 single knockdown were totally masked by those of miR-1/206 double knockdown. Although the reason for this needs further clarification, we suggested that miR-206 can directly regulate VegfAa protein level in somitic cells. In contrast, we further suggested that the miR-1 /SARS pathway may have the effect of fine-tuning angiogenesis, particularly as miR-1 must regulate the level of SARS protein before it can regulate the level of VegfAa ( Fig. 6 ). 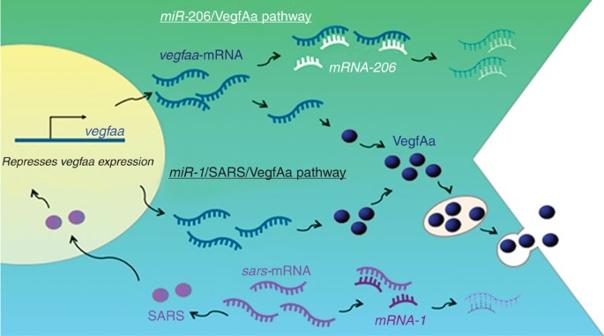Figure 6: Schematic representation showing the opposing roles played bymiR-1andmiR-206in the regulation of SARS and VegfAa. In somitic cells,miR-1serves as a pro-angiogenic modulator by inducing VegfAa expression through repressing SARS expression, whereasmiR-206serves as an anti-angiogenic modulator by directly repressingvegfaaexpression. These two pathways control the secreted levels of VegfAa from the somites to regulate angiogenesis. Figure 6: Schematic representation showing the opposing roles played by miR-1 and miR-206 in the regulation of SARS and VegfAa. In somitic cells, miR-1 serves as a pro-angiogenic modulator by inducing VegfAa expression through repressing SARS expression, whereas miR-206 serves as an anti-angiogenic modulator by directly repressing vegfaa expression. These two pathways control the secreted levels of VegfAa from the somites to regulate angiogenesis. Full size image miR-1 and miR-206 are evolutionarily conserved miRNA s of highly similar sequence. Their seed sequences are identical and their sequences outside the seed exist only four nt differences. As shown in Supplementary Fig. S4 , based on the theoretical prediction by bioinformatics analysis, the degree of complementarity between miR-1 and sars -3′UTR, as well as miR-206 and sars -3′UTR, is insignificant. However, based on in vivo experiments using luc assay in zebrafish embryos, as shown in Fig. 1e , we clearly demonstrated that simultaneous knockdown of miR-1 and miR-206 restores mt2 expression, but not individual knockdown of miR-1 or miR-206 . Meanwhile, mutated construct mt2 is targeted equally, or redundantly, by these two miRNAs , whereas mt3 is targeted specifically by miR-206 . Thus, we conclude that the endogenous sars -3′UTR target sequence (outside of seed) is refractory to miR-206 targeting, despite additional miR-206 complementarity. Instead, sars -3′UTR target sequence is specifically targeted by miR-1 . This result actually proved that the sequences in the neighbourhood of the seed are involved in the specificity of miRNA differential targeting, suggesting that the sequences outside the seed are critical for targeting selection. In addition that many principles for miRNA targeting, such as the local context of the target site can influence the efficiency of miRNA regulation [4] , [27] , the present study demonstrated that the two miRNA s with the same seed and strong similarities outside the seed do regulate different targets which provides important insight into new regulatory rules outside the seed in vivo . Many reports revealed that miR-1 is considered to be a tumour suppressor as overexpression of miR-1 can repress tumour growth [28] , [29] , [30] . However, other studies showed that miR-1 can induce cell proliferation and thus serve as an onco- miRNA in multiple myeloma plasma cell neoplasms [31] , [32] . Thus, the role of miR-1 in tumour growth might be cancer cell type-dependent because different cell lines express different Vegf-related miRNA s [33] . On the other hand, overexpression of miR-1/206 during muscle regeneration in rat can induce angiogenesis [17] . This result is consistent with the pro-angiogenic character of miR-1 , whereas, at the same time, it conflicts with the role of miR-206 . Angiogenesis is a crucial and delicate bioprocess from the standpoints of physiology and pathology, including development, regeneration, inflammation and tumour formation. As Vegf expression is a pivotal factor, it should be well regulated [34] , [35] . We hypothesized that VegfAa is variously regulated by miR-1/206 according to the cell type and physiological condition. We have shown that miR-1 and miR-206 have opposing roles in the regulation of vegfaa in somites during zebrafish embryogenesis ( Fig. 6 ). This contrasting functionality sheds more light on the complicated mechanisms underlying miRNA -modulated angiogenesis during embryonic development. Future studies will focus on the regulatory roles of miR-1 and miR-206 in angiogenesis under different physiological conditions, as well as the specific interactions between miR-1 / 206 and their target genes in terms of targeting mechanism and physiological relevance. Zebrafish husbandry and microscopy observation WT zebrafish ( Danio rerio ), transgenic lines Tg(fli1:EGFP) y1 (ref. 36 ) and Tg(fli1:nuclearEGFP) [37] provided by the Lawson’s Lab (UMASSMED) were maintained in aquaria according to standard procedures described by Westerfield [38] . The experiments and treatments of this animal have been reviewed and approved by the National Taiwan University Institutional Animal Care and Use Committee with ethics approval number: NTU-101-EL-115. Fluorescence was visualized with a fluorescent stereomicroscope (MZ FLIII, Leica) and a confocal spectral microscope (TCS SP5, Leica). MOs used to perform knockdown experiments The mRNAs were synthesized by the SP6 Message Machine Kit (Ambion). All MOs were purchased from Gene Tools (USA) and prepared according to the protocol published by Gene Tools. The sequence of the MOs we used were as follows: miR-1 -MO1 (AATACATACTTCTTTACATTCCA) [12] , miR-1 -MO2 (CATATGGGCATATAAAGAAGTATGT), miR206 -MO (GATCTCACTGAAGCCACACACTTCC), miR-1/206 -MO: (AGCCACACACTTCCTTACATTCCAT), sars -TP-MO (ACCTCTACTTGAAATATAGCACAAA), Control- MO (CCTCTTACCTCAGTTACAATTTATA), miR-1 -5mis-MO (AATA A ATA A TT G TTTA A ATT A CA), and miR-206 -5mis-MO (GAT A TCA A TGAA C CCA A ACA A TTCC) (the mismatched nt are underlined). Whole-mount in situ hybridization After we cloned the partial DNA fragments of the desired gene, the probes were Digoxigenin (DIG)-labelled. After permeabilization, embryos were hybridized overnight. Then, embryos were incubated with anti-DIG antibody (Roche; 1:8,000), stained and observed under a fluorescent stereomicroscope (MZ FLIII, Leica) [39] . To detect expression of mature miR-1 and miR-206 , DIG-labelled LNA probes were purchased from Integrated DNA technologies. The procedure of WISH was performed according to the protocol published by Exiqon. Western blot analysis Embryos were dechorionized, deyolked and lysed in whole-cell extract buffer (Hepes 20 mM; NaCl 0.2 M; TritonX100 0.5%; glycerol 20%; EDTA 1mM; and EGTA 1mM) containing the proteinase inhibitor cocktail (Roche). The lysates proteins were separated on SDS–PAGE and blotted with corresponding antibodies. The number of embryos used for each lane of gel ranged from 30 to 60 depending on the amount of examined proteins [39] , [40] . Antibodies against SARS (Abnova; H00006301-MO1; 25 μg ml −1 ; 1:1,000), GADPH (Santa Cruz; SC-32233; 100 μg ml −1 ; 1:1,000), α-tubulin (Sigma-Aldrich; T6199; 1 mg ml −1 ; 1:1,000), Vegfa (Abnova; MAB0294; 0.1 μg μl −1 ; 1:1,000), VegfAa (R & D; AF1247; 0.1 μg ml −1 ; 1:1,000), Anti-mouse-HRP (Santa Cruz; SC-2031; 200 μg per 0.5 ml; 1:5,000), and Anti-rabbit-HRP (Santa Cruz; SC-2004; 200 μg per 0.5 ml; 1:5,000) were used. Full scans of Western blots are shown in Supplementary Figs S8–S11 . Plasmid constructs The open reading frame (ORF) of sars from zebrafish (Z sars ) and mice (M sars ) were cloned from zebrafish embryos and mouse C2C12 cell line by PCR, respectively. The ORF of Z sars and M sars was, respectively, inserted into pCS2 + to generate pCS2 + -Z sars and pCS2 + -M sars , respectively. The pre- miR-1 and pre- miR-206 were cloned from zebrafish genomic DNA by PCR. The pre- miR-1 and pre- miR-206 were inserted into pCS2 + to generate pCS2 + - miR-1 and pCS2 + - miR-20 6. The 3′UTR of Z sars , M sars and Human sars (H sars ) were cloned from zebrafish embryos, mouse C2C12 cell line and Human HEK293T cell line. The 3′UTR of Z sars , M sars and H sars was, respectively, inserted into phRG-TK to generate phRG-TK-Z sars -3′UTR, phRG-TK-M sars -3′UTR and phRG-TK-H sars -3′UTR. The 3′UTR of Z sars was inserted into phRL- myf5 to generate phRL- myf5 -Z sars -3′UTR. In the in vivo luciferase experiment, we used PCR to mutate the miR-1 target sequences of Z sars -3′UTR, three mutated constructs were generated, as follows: Z sars -3′UTR-mt1 (ATAATTAACATTTGTGCTATATTTCA is mutated to ATAATTAACATTTGTGCTATAT AGGT ); Z sars -3′UTR-mt2 (ATAATTAACATTTGTGCTATATTTCA mutated to TATTAATTGTAAACACG TATATTTCA), and Z sars -3′UTR-mt3 (ATAATTAACATTTGTGCTATATTTCA mutated to CC AAT C AACATTTG C GCTATATTTCA). These mutated fragments were then inserted into phRL- myf5 to generate phRL- myf5 -Z sars -3′UTR-mt1, phRL- myf5 - Z sars -3′UTR-mt2 and phRL- myf5 -Z sars -3′UTR-mt3 individually. In the in vivo reporter experiment, the DNA fragments of Z sars -3′UTR and Z sars -3′UTR-mt1 were inserted into pCS2 + -EGFP to generate pCS2 + -EGFP-Z sars -3′UTR and pCS2 + -EGFP- Z sars -3'UTR-mt1, respectively. Non-canonical mutant SARS T429A SARS T429A is a SARS mutant whose canonical activity is blocked by the replacement of threonine located at 429 by Alanine (T429A), resulting in the inhibition of enzymatic activity that catalyses aminoacylation of transfer RNA for serine [14] . Although SARS T429A lacked canonical activity, it could still suppress the abnormal branching of ISVs in sars mutant fish (ko095) [14] . Following this logic, we used SARS T429A in this study to confirm whether the non-canonical activity of SARS is involved in miR-1 / 206 -mediated vascular development. Plasmids containing WT sars or sars mutant T429A were gifts from Prof. Kawahara (RIKEN [14] ). After the coding regions were amplified by PCR, the products were then inserted into pCS2 + expression vector to generate mRNAs in vitro using the mMESSAGE mMACHINE SP6 Kit (Ambion). Dual luciferase assay Dual luc reporter assay was carried out in cell lines HEK-293T and C2C12 following the standard protocol recommended by Promega with some modifications. In the control group, we co-transfected 20 ng of plasmid pGL3-TK, which served as an internal control, and 100 ng of each examined plasmid. In the experimental group, we cotransfected 20 ng of pGL3-TK, 100 ng of each examined plasmid plus 1.25 μg of plasmid pCS2 + - miR-1 or pCS2 + - miR-206. For dual luc reporter assay in zebrafish embryos, we coinjected 5 ng μl −1 of pGL3-TK, which also served as an internal control, and 5 ng μl −1 of phRL- myf5 , as described above, to serve as a control group, whereas we coinjected 5 ng μl −1 of pGL3-TK and 5 ng μl −1 of other luc reporter constructs to serve as an experimental group [41] . For each experiment, we randomly collected 30 embryos from 50 to 100 injected embryos and divided them into three groups ( n =10 per group) to carry out in vivo luciferase assays. Data for each experiment were the average of three groups. The final data, presented as mean±s.d., were an average of three independent experiments, which were carried out on different days. Enzyme-linked immunosorbent assay The supernatants collected from C2C12 cells transfected separately with miR-1 and M sars for 48 h were assayed using an ELISA kit for mVegf (eBioscience) according to the manufacturer’s instructions. qPCR For each experiment, we collected 100 embryos in 500 ml of Trizol Reagent (Invitrogen). Total RNAs were isolated according to the manufacturer’s instructions. For qPCR, first-strand cDNA was generated using 1 mg of total RNA. Both cDNA concentrations were adjusted to 200 ng ml −1 , and qPCR was performed using the 7900HT Fast Real-Time PCR System (Applied Biosystems) according to the manufacturer’s instructions. Forward and reverse primers describe by Fukui et al. [14] were used, as follows: forward primer TCCTGTGTGGTTCTCATGC and reverse primer TGCATTCACACTTGGTGTGTTC for amplifying zebrafish vegfaa ; forward primer CTCCTCTTGGTCGCTTTGCT and reverse primer CCGATTTTCTTCTCAACGCTCT for amplifying ef1a. Expression levels were determined by comparison with a standard curve from total RNAs isolated from WT embryos. For quantitative detection of miR-1 and miR-206 in embryos at 12, 16, 20, 24, 28 and 32 hpf, the cDNAs of miR-1 and miR-206 were synthesized by miR-1 -RT primer (CTCAACTGGTGTCGTGGAGTCGGCAATTCAGTTGAGATACAT) and miR-206 -RT primer (CCATCATGCTCTCGACCTGTCCGATCACGACGAGAGCATGATGGCCACAC). For qPCR of miR-1 , the primers were miR-1 -F (GCTATGGAATGTAAAGAAGTATGTAT) and miR-1 -R (CTCAACTG- GTGTCGTGGAGTC). For qPCR of miR-206 , the primers were miR-206 -F (GTTATGGAATGTAAGGAAGTGTGTGG) and miR-206 -R (CCATCATGCTCTCGACCTGTC). The internal controls for miR-1 and miR-206 were β-actin (β-actin-1072F:GGATCGGTGGCTCCATCTT; β-actin -1144R:TCATCGTACTC- CTGCTTGCTGAT) and EF1α ( EF1α -1330F: CTCCTCTTGGTCGCTTTGCT; EF1α -1411R: CCGATTTTCTTCTCAACGCTCT). To compare the relative expression levels of miR-1 and miR-206 at each stage, the expression levels of miR-1 and miR-206 at 12 hpf were set as 1. To determine the copy number of miR-1 and miR-206, zebrafish U6 snRNA was used as endogenous control. Specific plasmids were constructed for miR-1 , miR-206 and U6 by cloning products for real-time PCR. Knowing the size of the plasmid that contains the gene of interest, the number of grams/molecule and copy number can be calculated as follows: Weight in Daltons (g mol −1 )=(bp of double-stranded product) × (330 Da × 2nt per bp). Hence, (g mol −1 )/Avogadro’s number= g per molecule=copy number. Knowing the copy number and concentration of plasmid DNA, the precise number of molecules added to subsequent real-time PCR can be calculated, thus providing a standard for specific cDNA quantification. Real-time PCR was carried out in a MicroAmp Optical 96-well plate using power SYBR Green PCR Master Mix (Applied Biosystems), with 2 μl cDNA or Specific control DNA (10 2 –10 6 copies) in each well. PCR reactions were monitored in real time using the ABI 7900HT Fast Real-time PCR system (Applied Biosystems). The thermal cycling conditions for real-time PCR were 50 °C for 2 min, then 95 °C for 10 min and 40 cycles of denature (95 °C, 15 s) and annealing/extension (60 °C, 60 s). A standard curve was drawn by plotting the natural log of the threshold cycle (CT) against the natural log of the number of molecules. CT was calculated under default settings for real-time sequence detection software (Applied Biosystems). The equation drawn from the graph was used to calculate the precise number of specific cDNA molecules tested in the same reaction plate as the standard. For qPCR of U6, the primers were U6-F (ACTAAAATTGGAACGATACAGAGA) and U6-R (AAAGATGGAACGCTTCACG). To compare the relative expression levels of miR-1 and miR-206 at each stage, the expression levels of miR-1 and miR-206 which normalized to U6 at 12 hpf were set as 1. Statistical analysis Data were averaged from three independent experiments and presented as mean±s.d., and difference levels were analysed using Student’s t -test. * P <0.05, ** P <0.01 and *** P <0.005 indicated the significant difference levels. How to cite this article: Lin, C.-Y. et al. miR-1 and miR-206 target different genes to have opposing roles during angiogenesis in zebrafish embryos. Nat. Commun. 4:2829 doi: 10.1038/ncomms3829 (2013).